Kinetochores require oligomerization of Dam1 complex to maintain microtubule attachments against tension and promote biorientation Kinetochores assemble on centromeric DNA and present arrays of proteins that attach directly to the dynamic ends of microtubules. Kinetochore proteins coordinate at the microtubule interface through oligomerization, but how oligomerization contributes to kinetochore function has remained unclear. Here, using a combination of biophysical assays and live-cell imaging, we find that oligomerization of the Dam1 complex is required for its ability to form microtubule attachments that are robust against tension in vitro and in vivo . An oligomerization-deficient Dam1 complex that retains wild-type microtubule binding activity is primarily defective in coupling to disassembling microtubule ends under mechanical loads applied by a laser trap in vitro . In cells, the oligomerization-deficient Dam1 complex is unable to support stable bipolar alignment of sister chromatids, indicating failure of kinetochore–microtubule attachments under tension. We propose that oligomerization is an essential and conserved feature of kinetochore components that is required for accurate chromosome segregation during mitosis. Accurate chromosome segregation is mediated by kinetochores, which physically link replicated chromosomes to the bipolar mitotic spindle. During mitosis, kinetochores utilize microtubule tip dynamics to produce mechanical forces required for chromosome biorientation and segregation. In the budding yeast Saccharomyces cerevisiae , the heterodecameric Dam1 complex is responsible for coupling kinetochores to microtubule ends and for maintaining these attachments during biorientation, when tension is applied across the kinetochores assembled on sister chromatid pairs [1] , [2] , [3] . In vitro , the Dam1 complex spontaneously assembles into oligomeric rings that encircle microtubules, and it has long been hypothesized that the ability to adopt this ring conformation is critical for its roles in kinetochore–microtubule attachment [4] , [5] , [6] , [7] . However, ring formation is not required for the Dam1 complex to track with disassembling microtubule ends in the absence of applied tension in vitro [8] . Thus, it remains unclear whether oligomerization is required for any specific functions of the Dam1 complex, or even if oligomeric rings exist at kinetochores during mitosis. The Dam1 complex is required for kinetochores to sustain attachments to microtubule ends against high forces, and to modify microtubule tip dynamics to promote microtubule growth [9] , [10] , [11] . It binds to kinetochores via direct interaction with the Ndc80 complex on microtubules [12] , [13] . Here to address whether oligomerization is important for any of these functions, we used a Dam1 subcomplex that lacks the ability to assemble into oligomeric rings on microtubules, as determined by negative-stain electron microscopy [14] . Deletion of the gene encoding Hsk3 causes the remaining nine components of the Dam1 complex to split into two subcomplexes. One of these contains six proteins—Dam1, Duo1, Spc34, Spc19, Dad1 and Dad3—and binds microtubules in vitro . This is the ‘Oligomerization-Deficient’ Dam1 OD complex used in this study. The other three components (Ask1, Dad2 and Dad4) form the second subcomplex, which does not bind microtubules [14] . Using in vitro biochemical and biophysical assays, we found that the Dam1 OD complex represents a clean separation of functions: it retains an intact microtubule-binding site, but is deficient in oligomerization. We identified a striking defect of the Dam1 OD complex in coupling to disassembling microtubule tips against applied tension. Finally, we asked if oligomerization of the Dam1 complex is required in vivo . As every component of the Dam1 complex is essential for viability [15] , an Hsk3–degron system was used to transiently generate the Dam1 OD complex in yeast cells. Consistent with our in vitro observations, kinetochore–microtubule attachments in these cells failed during bipolar alignment of sister chromatids, resulting in mitotic arrest. Our work provides compelling evidence for a specific and essential function of oligomerization at the kinetochore–microtubule interface. Microtubule binding and oligomerization are separable Miranda et al . [14] previously reported a stable, six-protein Dam1 subcomplex that co-sediments with microtubules, but is unable to assemble into oligomeric rings ( Supplementary Fig. 1 ). We corroborated and expanded these findings to verify the fact that this Oligomerization-Deficient Dam1 OD complex retains a functional microtubule-binding domain in the absence of oligomerization. Using total internal reflection fluorescence (TIRF) microscopy [8] , [12] , we imaged single wild-type (Dam1 WT ) and Dam1 OD complexes tagged with Dad1–green fluorescent protein (GFP) as they bound to microtubules ( Fig. 1a ). Distributions of GFP fluorescence intensity were similar for the Dam1 WT and Dam1 OD complexes, and the magnitude of single photobleach steps in our imaging conditions suggests that these distributions derive from single GFP molecules ( Fig. 1b ). Thus, at the low concentrations (5–40 pM) required for single-molecule imaging, both Dam1 WT and Dam1 OD complexes exist primarily as monomers. Residence time distributions and standard diffusion plots showed that the Dam1 WT and Dam1 OD complexes exhibit similar microtubule-binding properties ( Fig. 1c,d ). We determined single-molecule mean residence times of 5.3±0.5 (error of the mean) and 7.0±0.5 s, and diffusion constants of 0.021±0.001 (s.d. of the fit) and 0.017±0.001 μm 2 s −1 , for Dam1 WT and Dam1 OD complexes, respectively. Thus, at the single-molecule level, the oligomerization-deficient Dam1 complex binds microtubules in a manner that is similar to the wild-type (WT) complex. 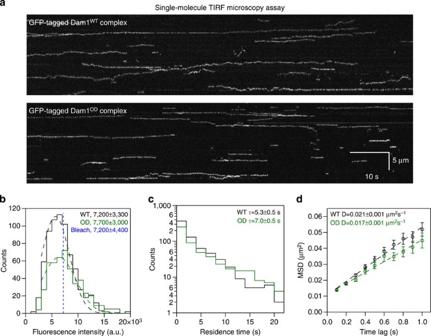Figure 1: The oligomerization-deficient Dam1 complex retains an intact microtubule-binding site. (a) Kymographs show single molecules of GFP-tagged wild-type (top) and oligomerization-deficient (bottom) Dam1 complex as they bound to and diffused along taxol-stabilized microtubules. Scale bar applies to both kymographs; image brightness and contrast were adjusted identically. (b) Histograms of GFP brightness intensity for single molecules of wild-type (WT, black trace,n=717) and oligomerization-deficient (OD, green trace,n=472) Dam1 complex on microtubules. Dashed-blue line indicates the average height of single-step photobleaches under identical imaging conditions (n=295). Brightness values are reported as mean±s.d. (c) Residence time distributions for individual Dam1WT(n=717) and Dam1OD(n=564) complexes on microtubules. Mean residence time,τ±error of the mean was estimated by bootstrapping analysis (see Methods for additional details). (d) Mean-squared displacement (MSD) versus time lag for single particles (WT,n=654; OD,n=506) represented incandd. Error bars on each point indicate s.e.m. Dashed lines indicate weighted linear fits to the data, yielding the diffusion constants, D±s.d. of the fit. Figure 1: The oligomerization-deficient Dam1 complex retains an intact microtubule-binding site. ( a ) Kymographs show single molecules of GFP-tagged wild-type (top) and oligomerization-deficient (bottom) Dam1 complex as they bound to and diffused along taxol-stabilized microtubules. Scale bar applies to both kymographs; image brightness and contrast were adjusted identically. ( b ) Histograms of GFP brightness intensity for single molecules of wild-type (WT, black trace, n =717) and oligomerization-deficient (OD, green trace, n =472) Dam1 complex on microtubules. Dashed-blue line indicates the average height of single-step photobleaches under identical imaging conditions ( n =295). Brightness values are reported as mean±s.d. ( c ) Residence time distributions for individual Dam1 WT ( n =717) and Dam1 OD ( n =564) complexes on microtubules. Mean residence time, τ ±error of the mean was estimated by bootstrapping analysis (see Methods for additional details). ( d ) Mean-squared displacement (MSD) versus time lag for single particles (WT, n =654; OD, n =506) represented in c and d . Error bars on each point indicate s.e.m. Dashed lines indicate weighted linear fits to the data, yielding the diffusion constants, D±s.d. of the fit. Full size image At a higher concentration (2 nM) that supports the formation of oligomeric rings [12] , Dam1 WT complex formed a punctate distribution along microtubules, consistent with its cooperative binding [8] and its assembly into oligomers ( Supplementary Fig. 2a ). Despite their similar behaviour at the single-molecule level, 2 nM Dam1 OD complex decorated the microtubule lattice at a much lower density relative to 2 nM Dam1 WT complex ( Supplementary Fig. 2b ). Instead, 20 nM Dam1 OD complex was needed to achieve a binding density on microtubules comparable to that of 2 nM WT, and the decoration by Dam1 OD complex appeared more uniform ( Supplementary Fig. 2a,b ). Thus, the Dam1 OD complex is impaired in binding cooperativity, as expected for an oligomerization-deficient species. We visualized individual molecules in these conditions by mixing small (‘tracer’) quantities of GFP-tagged Dam1 complex with excess un-tagged complex ( Supplementary Fig. 2c–e ). For Dam1 WT complex, ‘tracer’ GFP-tagged molecules exhibited long residence times on the microtubule lattice, suggesting their incorporation into oligomers of un-tagged Dam1 WT complexes ( Supplementary Fig. 2c ). We note that the residence time of ‘tracer’ Dam1 WT complexes, 56±8 s ( Supplementary Fig. 2f ), is comparable to the average single-step photobleaching time in our imaging conditions (51±16 s). Therefore, this measurement likely underestimates the lifetime of oligomeric assemblies of Dam1 WT complex on microtubules. By contrast, ‘tracer’ Dam1 OD complexes were unaffected by the addition of excess un-tagged Dam1 OD complex. The residence time for ‘tracer’ Dam1 OD complexes was 7.0±0.6 s ( Supplementary Fig. 2d,f ), indistinguishable from the residence time in the absence of excess un-tagged Dam1 OD complexes, 7.0±0.5 s ( Fig. 1c ). Thus, the Dam1 OD complex does not form stable oligomers on microtubules. Interestingly, the mean residence time of ‘tracer’ Dam1 OD complexes increased 1.8-fold (12.5±1.2 s) in the presence of excess unlabeled Dam1 WT complexes, indicating that the Dam1 OD complex can associate with the Dam1 WT complex ( Supplementary Fig. 2e,f ). Because the residence time is only doubled, the OD complex must only associate with one or a few Dam1 WT complexes and does not form rings. Finally, by combining gel filtration and velocity sedimentation analyses, we estimated the molecular weight of the Dam1 WT and Dam1 OD complexes to assess oligomerization state in solution. Even at concentrations above 1 μM, the Dam1 OD complex is monomeric in solution ( Supplementary Fig. 3 ), while the Dam1 WT complex exists primarily as a dimer, as reported previously [12] , [16] . Unlike the Dam1 WT complex, the Dam1 OD complex does not dimerize in solution or homo-oligomerize on microtubules. However, the microtubule-binding site of the Dam1 OD complex appears intact at the single-molecule level and behaves similar to a single Dam1 WT complex. Therefore, the interfaces that mediate microtubule-binding and oligomerization are contained in structurally distinct modules within the Dam1 complex. These modules can be separated to measure how oligomerization contributes to kinetochore–microtubule attachment in vitro and in vivo . Oligomerization is required for the strongest attachments An optical trap-based rupture force assay [12] , [17] was used to assess the strength of microtubule attachments mediated by the WT Dam1 complex and by the oligomerization-deficient complex ( Fig. 2a,b ). Dam1 complexes were loaded onto polystyrene beads at relatively high surface density to promote the formation of oligomers, such that up to ~80 individual complexes could simultaneously interact with the microtubule tip [18] . Beads coated with Dam1 OD complexes yielded a median rupture force similar to that for beads coated with Dam1 WT complexes (4.8 and 5.2 pN, respectively). However, there is an extended ‘tail’ on the distribution for Dam1 WT complex at very high rupture forces; this tail is absent for the Dam1 OD complex ( Fig. 2c , Table 1 ). The maximum rupture force observed for Dam1 WT complex, 15.2 pN, is almost twofold higher than that for the Dam1 OD complex, 8.3 pN. This was not an isolated instance, as 13% of all ruptures for Dam1 WT complex occurred above the maximum rupture force for the Dam1 OD complex ( Fig. 2c ). These findings suggest that oligomerization is required for the formation of strong microtubule attachments. 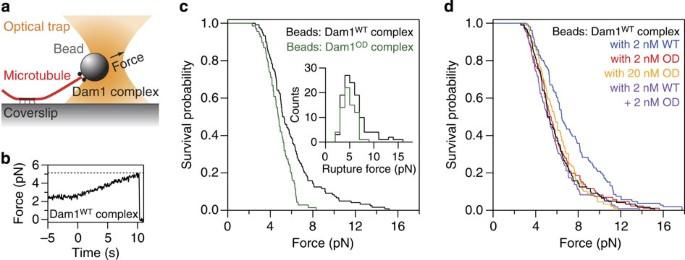Figure 2: Oligomerization of the Dam1 complex enhances microtubule attachment strength. (a) Diagram of the optical trap assay. (b) Example trace of applied force versus time from the rupture force assay. Beads are subjected to a ~2.5-pN test force prior to initiation of the force ramp (~0.25 pN s−1), which begins att=0 s. Dashed line indicates the rupture force from this event. (c) Survival versus force curves for beads coated with wild-type (WT, black trace,n=120) or oligomerization-deficient (OD, green trace,n=69) Dam1 complexes coupled to microtubule tips. Inset: same data represented in survival curves but re-plotted as rupture force histograms. (d) Survival versus force curves for beads coated with Dam1WTcomplex alone (black trace, reproduced fromc) or in the presence of additional Dam1 complex free in solution: with 2 nM Dam1WTcomplex, blue,n=106; with 2 nM Dam1ODcomplex, red,n=86; with 20 nM Dam1ODcomplex, orange,n=89; with 2 nM Dam1WTand 2 nM Dam1ODcomplex, purple,n=109. Figure 2: Oligomerization of the Dam1 complex enhances microtubule attachment strength. ( a ) Diagram of the optical trap assay. ( b ) Example trace of applied force versus time from the rupture force assay. Beads are subjected to a ~2.5-pN test force prior to initiation of the force ramp (~0.25 pN s −1 ), which begins at t =0 s. Dashed line indicates the rupture force from this event. ( c ) Survival versus force curves for beads coated with wild-type (WT, black trace, n =120) or oligomerization-deficient (OD, green trace, n =69) Dam1 complexes coupled to microtubule tips. Inset: same data represented in survival curves but re-plotted as rupture force histograms. ( d ) Survival versus force curves for beads coated with Dam1 WT complex alone (black trace, reproduced from c ) or in the presence of additional Dam1 complex free in solution: with 2 nM Dam1 WT complex, blue, n =106; with 2 nM Dam1 OD complex, red, n =86; with 20 nM Dam1 OD complex, orange, n =89; with 2 nM Dam1 WT and 2 nM Dam1 OD complex, purple, n =109. Full size image Table 1 The rupture force assay reveals how oligomerization of the Dam1 complex contributes to microtubule attachment strength. Full size table To further investigate this hypothesis, we performed the rupture force assay in the presence of additional Dam1 complex added free in solution. By design of the assay, free Dam1 complex was unable to load directly onto the bead surface, and could only affect attachment strength by oligomerizing with bead-bound Dam1 complex. Relative to Dam1 WT complex on the beads alone, the addition of 2 nM free Dam1 WT complex significantly increased the proportion of strong attachments ( Fig. 2d , Table 1 ): the median rupture force increased to 6.5 pN, and 30% of all ruptures occurred at high force (above 8.3 pN). In contrast, the behaviour of Dam1 WT complex on beads was not enhanced by the addition of free Dam1 OD complex ( Fig. 2d ), even when 10-fold more was added to compensate for its decreased microtubule decoration seen by TIRF microscopy. Based on our observation that the Dam1 OD and Dam1 WT complexes can interact directly, we further reasoned that free Dam1 OD complex might interfere with oligomerization by the Dam1 WT complex. Indeed, the enhancement in strength afforded by free Dam1 WT complex was completely negated by simultaneous addition of free Dam1 OD complex in solution ( Fig. 2d ). Therefore, we propose that the Dam1 OD complex acts as a competitive inhibitor in the rupture force assay by ‘capping’ Dam1 WT oligomers. Our results demonstrate that oligomers of Dam1 complex are necessary to sustain microtubule attachments against high forces. Oligomerization is not required to bind kinetochores In vivo , the Ndc80 to complex is required for the Dam1 complex to associate with kinetochores, which occurs after initial kinetochore capture on the lateral face of spindle microtubules [2] , [3] , [13] . The Dam1 complex promotes kinetochore–microtubule attachment strength and is required for maturation of these attachments from lateral to end-on [1] , [2] . Using the optical trap-based rupture force assay, we tested if the Dam1 complex must oligomerize to bind the Ndc80 complex and strengthen its attachment to microtubules. As previously reported [12] , the Ndc80 complex formed weak microtubule attachments (mean rupture force: 2.5±0.2 pN, error indicates s.e.m.) that were greatly enhanced by the addition of the Dam1 WT complex (7.4±0.4 pN) free in solution ( Fig. 3a , Table 1 ). The Dam1 OD complex also strengthened Ndc80-based attachments (4.8±0.2 pN), albeit to a lesser extent than WT ( Fig. 3a , Table 1 ). We further asked if the Dam1 OD complex could bind to native kinetochore particles isolated from budding yeast, and strengthen their attachments to microtubules in vitro . To inactivate endogenous Dam1 complex, kinetochore particles were purified from cells carrying the temperature-sensitive dad1-1 mutation after being shifted to the restrictive temperature. Consistent with previous work [10] , [11] , WT kinetochore particles yielded a mean rupture force of 9.7±1.0 pN, while dad1-1 kinetochores were much weaker at 2.7±0.2 pN ( Fig. 3b , Table 1 ). The mean rupture force of dad1-1 kinetochores was partially rescued by the addition of Dam1 WT complex to 5.6±0.3 pN ( Fig. 3b , Table 1 ). The Dam1 OD complex was less effective but still partially rescued attachment strength to 3.7±0.2 pN ( Fig. 3b , Table 1 ). Thus, oligomerization is not strictly required for the Dam1 complex to transmit load to the kinetochore through the Ndc80 complex. 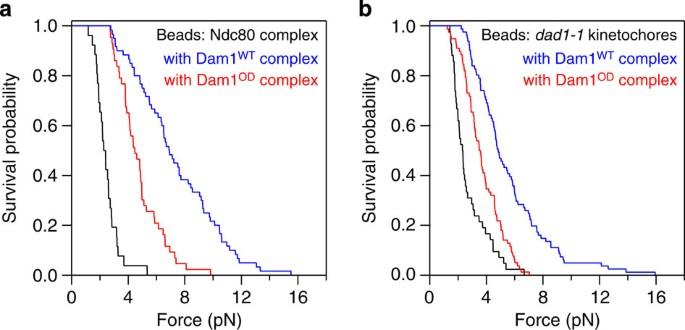Figure 3: The Dam1 complex loads onto kinetochores in the absence of oligomerization. (a) Survival versus force curves for beads coated with Ndc80 complex alone (black trace,n=26) or in the presence of free wild-type (WT, blue trace,n=60) or oligomerization-deficient (OD, red trace,n=43) Dam1 complex in solution. (b) As ina, using beads instead coated with purified kinetochore particles lacking functional endogenous Dam1 complex (dad1-1kinetochores). Beads were assayed alone (black trace,n=42), and in the presence of purified, recombinant Dam1WT(blue trace,n=81) or Dam1OD(red trace,n=78) complex added free in solution. Figure 3: The Dam1 complex loads onto kinetochores in the absence of oligomerization. ( a ) Survival versus force curves for beads coated with Ndc80 complex alone (black trace, n =26) or in the presence of free wild-type (WT, blue trace, n =60) or oligomerization-deficient (OD, red trace, n =43) Dam1 complex in solution. ( b ) As in a , using beads instead coated with purified kinetochore particles lacking functional endogenous Dam1 complex ( dad1-1 kinetochores). Beads were assayed alone (black trace, n =42), and in the presence of purified, recombinant Dam1 WT (blue trace, n =81) or Dam1 OD (red trace, n =78) complex added free in solution. Full size image Robust coupling against tension requires oligomerization At the kinetochore, the Dam1 complex enhances the strength and processivity of microtubule linkages [12] , [13] . Stable kinetochore–microtubule coupling is crucial when chromosomes become bioriented by the mitotic spindle, as tension is applied across sister kinetochore pairs. It has long been hypothesized that oligomerization is required for the Dam1 complex to support robust coupling to dynamic microtubule ends against applied mechanical loads [4] , [5] . To test this hypothesis, we programmed the laser trap to apply constant force against Dam1 complexes as they coupled beads to dynamic microtubule tips [9] , [19] . When linked directly to beads, both Dam1 WT and Dam1 OD complexes were able to maintain attachments for assembling microtubule tips over the course of several minutes (9.9±1.9 min and 2.8±0.3 min, respectively; error is estimated from counting statistics) against a constant load of 2.4 pN ( Fig. 4a ). During this time, the Dam1 WT and Dam1 OD complexes had similar effects on microtubule dynamics. Microtubule tips exhibited similar average rates of growth and catastrophe, the transition from assembly to disassembly ( Fig. 4b,c ). Following catastrophe events, beads coated with Dam1 WT complex coupled to disassembling microtubules for 1.0±0.3 min against the applied force. Furthermore, Dam1 WT complex slowed the rate of microtubule disassembly and promoted rescue (the transition from shortening to growth), as previously reported [9] ( Fig. 4b,c ). By contrast, beads decorated with Dam1 OD complex failed to couple robustly for disassembling tips against force, as evidenced by their detachment within 0.05±0.01 min (3 s) on average ( Fig. 4a ). Dam1 OD complex also regulated disassembly speed less effectively, and we were unable to observe any rescue events due to the short lifetime of these attachments ( Fig. 4b,c ). Importantly, the Dam1 OD complex was impaired in disassembly-driven motility only when acting against an applied force. In the absence of force, every bead tested ( n =15) underwent processive tracking with a disassembling microtubule end. Most beads (13 of 15) tracked disassembly all the way to the stabilized microtubule seed, while only two events ended in detachment, yielding a mean lifetime of ~5 min during disassembly in the absence of force. Thus, the oligomerization-deficient Dam1 complex is strikingly defective in coupling to and regulating the dynamics of disassembling microtubule tips under load. 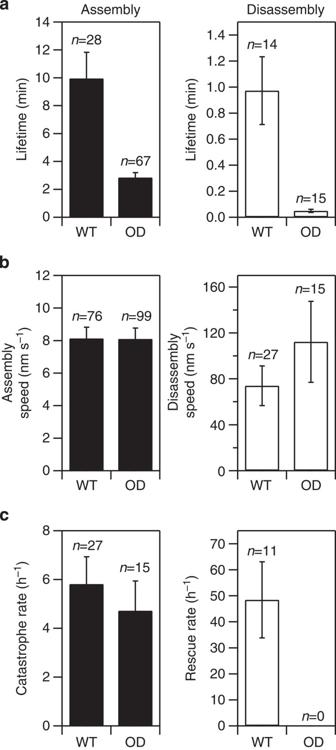Figure 4: The oligomerization-deficient Dam1 complex fails to track with disassembling microtubule tips against applied load. Beads coated with wild-type (WT) or oligomerization-deficient (OD) Dam1 complex were tracked while they coupled to assembling (left plots) and disassembling (right plots) microtubule tips under a constant force of ~2.4 pN applied in the direction of microtubule assembly. (a) Mean attachment lifetime for beads coupled to dynamic microtubule tips under constant load. (b) Speeds of microtubule tip assembly and disassembly while coupled to beads under constant force. In our assay conditions, the intrinsic rates of microtubule assembly and disassembly are ~6 nm s−1and ~230 nm s−1, respectively9,34. (c) Switch rates for microtubule tip state: from assembly to disassembly (catastrophe), and from disassembly to assembly (rescue). For microtubules alone, catastrophes occur at a frequency of ~10 h−1(refs9,45), and rescues at ~2 h−1(ref.34). Ina–c, error bars indicate s.e.m. Figure 4: The oligomerization-deficient Dam1 complex fails to track with disassembling microtubule tips against applied load. Beads coated with wild-type (WT) or oligomerization-deficient (OD) Dam1 complex were tracked while they coupled to assembling (left plots) and disassembling (right plots) microtubule tips under a constant force of ~2.4 pN applied in the direction of microtubule assembly. ( a ) Mean attachment lifetime for beads coupled to dynamic microtubule tips under constant load. ( b ) Speeds of microtubule tip assembly and disassembly while coupled to beads under constant force. In our assay conditions, the intrinsic rates of microtubule assembly and disassembly are ~6 nm s −1 and ~230 nm s −1 , respectively [9] , [34] . ( c ) Switch rates for microtubule tip state: from assembly to disassembly (catastrophe), and from disassembly to assembly (rescue). For microtubules alone, catastrophes occur at a frequency of ~10 h −1 (refs 9 , 45 ), and rescues at ~2 h −1 (ref. 34 ). In a – c , error bars indicate s.e.m. Full size image Oligomerization is important for biorientation in vivo Based on our in vitro results, we predicted that the oligomerization-deficient Dam1 complex should localize to kinetochores and bind microtubules in vivo , but fail to mediate kinetochore–microtubule attachments against the forces experienced during biorientation. Since deletion of HSK3 is lethal in budding yeast [20] , [21] , we targeted Hsk3 with an inducible degron system [22] to transiently generate the Dam1 OD complex in vivo ( Supplementary Fig. 4a,b ). Degron induction caused cells to arrest with large buds, indicating mitotic arrest and suggesting an essential role for Hsk3 during mitosis. Localization of the two structural modules of the Dam1 complex was tracked in Hsk3-depleted cells using Dad1–GFP (in the microtubule-binding module) and Ask1–yellow fluorescent protein (YFP) (in the oligomerization module). Consistent with the formation of the Dam1 OD complex in vivo , depletion of Hsk3 decoupled the localization of these two modules. Dad1–GFP retained localization to kinetochores and the mitotic spindle similar to control cells, while Ask1–YFP became delocalized ( Fig. 5a,b and Supplementary Fig. 4c,d ). To verify that this is a specific outcome of depleting Hsk3, rather than a generic result of disrupting the Dam1 complex, we targeted the degron system to the Dam1 protein ( Supplementary Fig. 5a,b ). Depletion of Dam1 caused both Dad1–GFP and Ask1–YFP to delocalize ( Fig. 5c and Supplementary Fig. 5c,d ). These findings suggest that the Hsk3–degron system generates a stable Dam1 OD complex in vivo and does not simply disrupt the entire Dam1 complex. 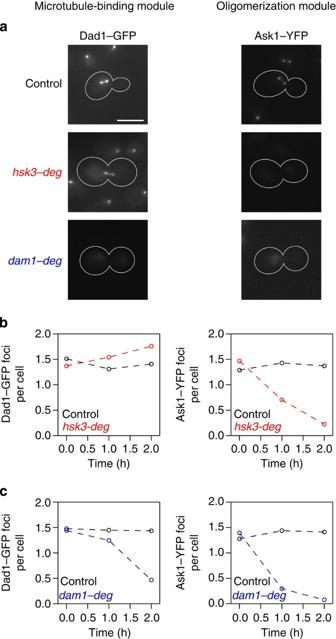Figure 5: Depletion of Hsk3 causes formation of the oligomerization-deficient Dam1 complexin vivo. (a) Representative images of Dad1–GFP and Ask1–YFP in mitotic control (top),hsk3–degron(middle) anddam1–degron(bottom) cells at 2 h after addition of auxin. Scale bar is 5 μm and applies to all images. Localization of Dad1–GFP (b) and Ask1–YFP (c) was quantified by automated spot detection and is reported as the average number of detected foci per cell. For both Dad1–GFP and Ask1–YFP, asynchronously growing cells have ~1.4 foci per cell on an average, indicating a mix of mitotic (2 foci) and non-mitotic (1 focus) cells. Arrest in mitosis with kinetochore localization causes the average to approach 2.0 foci per cell; delocalization is indicated by a trend towards 0 foci per cell. SeeSupplementary Figs 3 and 4for the number of cells counted in each condition. Figure 5: Depletion of Hsk3 causes formation of the oligomerization-deficient Dam1 complex in vivo . ( a ) Representative images of Dad1–GFP and Ask1–YFP in mitotic control (top), hsk3–degron (middle) and dam1–degron (bottom) cells at 2 h after addition of auxin. Scale bar is 5 μm and applies to all images. Localization of Dad1–GFP ( b ) and Ask1–YFP ( c ) was quantified by automated spot detection and is reported as the average number of detected foci per cell. For both Dad1–GFP and Ask1–YFP, asynchronously growing cells have ~1.4 foci per cell on an average, indicating a mix of mitotic (2 foci) and non-mitotic (1 focus) cells. Arrest in mitosis with kinetochore localization causes the average to approach 2.0 foci per cell; delocalization is indicated by a trend towards 0 foci per cell. See Supplementary Figs 3 and 4 for the number of cells counted in each condition. Full size image To ask if oligomerization is required for normal kinetochore–microtubule attachment, cells were depleted of Hsk3 and imaged as they entered mitosis. Upon separation of the duplicated spindle pole bodies, kinetochores (marked by Nuf2–GFP) in control cells aligned symmetrically between the two spindle poles, while in Hsk3-depleted cells, kinetochores often aligned asymmetrically towards one pole ( Fig. 6a–c ). Hsk3-depleted cells additionally exhibited abnormal spindle lengths (for example, Fig. 6b shows spindle hyper-extension), consistent with the high incidence of spindle breakage observed in an extended degron-induced arrest ( Supplementary Fig. 6 ). Asymmetric kinetochore clustering towards one pole is inconsistent with a lack of kinetochore–microtubule attachment, which causes unclustering of kinetochores in the nucleus [23] , [24] , [25] , [26] . Instead, this asymmetric kinetochore clustering phenotype suggests a defect in sister kinetochore biorientation [3] , [27] . To quantify asymmetry in the kinetochore distribution, we developed a ‘kinetochore intensity ratio’ metric. Nuf2–GFP fluorescence intensity was integrated across the two halves of each spindle ( Fig. 6a,b ), and a ratio was taken of the brighter side over the dimmer side (and is thus always ≥1). For control cells, this ratio was narrowly distributed around the average of 1.1±0.02 (s.e.m. ), indicating accurate bipolar segregation of kinetochores with high fidelity ( Fig. 6d,e ). By contrast, kinetochore intensity ratios for Hsk3-depleted cells varied widely (from 1.0 to 14) and averaged 3.3±0.6, reflecting a strong bias towards monopolar alignment that was evident across all observed spindle lengths ( Fig. 6d,e ). Therefore, the equal partitioning of kinetochores during mitosis requires oligomerization of the Dam1 complex. 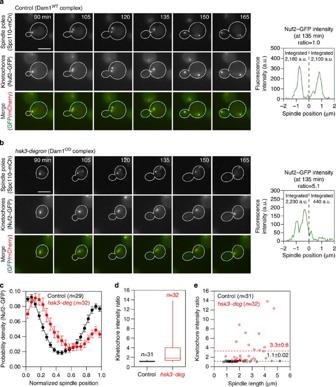Figure 6: Equal bipolar distribution of kinetochores requires oligomerization of the Dam1 complex. Time-lapse images of spindle poles (Spc110–mCherry, top row), kinetochores (Nuf2–GFP, middle row) and merged channels (bottom row) in control (a) andhsk3–degron(b) cells. Cells were imaged immediately following release from α-factor (G1) arrest; time stamps show time after release. Scale bars, 5 μm. At right in bothaandbare spindle profiles of Nuf2–GFP intensity from corresponding images taken at 135 min after release. The integrated intensity in each half-spindle is printed on the plot. (c) Average spindle intensity profiles of Nuf2–GFP in control (black curve) andhsk3–degron(red curve) cells. Markers indicate average±s.e.m. (d) Box and whisker plots show the distribution of kinetochore intensity ratios measured for control andhsk3–degroncells. Whiskers show the full range of the distribution, while the box shows the 75th, 50th and 25th percentiles. (e) Plot of kinetochore intensity ratio versus spindle length shows that asymmetric kinetochore alignment inhsk3–degroncells is independent of spindle length. See Methods for additional information about the measurements presented in this figure. Figure 6: Equal bipolar distribution of kinetochores requires oligomerization of the Dam1 complex. Time-lapse images of spindle poles (Spc110–mCherry, top row), kinetochores (Nuf2–GFP, middle row) and merged channels (bottom row) in control ( a ) and hsk3–degron ( b ) cells. Cells were imaged immediately following release from α-factor (G1) arrest; time stamps show time after release. Scale bars, 5 μm. At right in both a and b are spindle profiles of Nuf2–GFP intensity from corresponding images taken at 135 min after release. The integrated intensity in each half-spindle is printed on the plot. ( c ) Average spindle intensity profiles of Nuf2–GFP in control (black curve) and hsk3–degron (red curve) cells. Markers indicate average±s.e.m. ( d ) Box and whisker plots show the distribution of kinetochore intensity ratios measured for control and hsk3–degron cells. Whiskers show the full range of the distribution, while the box shows the 75th, 50th and 25th percentiles. ( e ) Plot of kinetochore intensity ratio versus spindle length shows that asymmetric kinetochore alignment in hsk3–degron cells is independent of spindle length. See Methods for additional information about the measurements presented in this figure. Full size image To directly test for a defect in sister kinetochore biorientation, we visualized individual sister centromere pairs in Hsk3-depleted cells. Consistent with the asymmetric distribution of kinetochores, the majority of Hsk3-depleted cells (83%) had a monopolar CEN3 pair, while only 17% contained a CEN3 pair in a bipolar state ( Fig. 7 ). Of the bipolar CEN3 pairs, 31% collapsed to monopolar attachments within 30 min of observation ( Fig. 7c and Supplementary Fig. 7 ). These events provide direct evidence for microtubule attachment failure by one kinetochore of the sister pair. In control cells, weak or erroneous attachments were rarely observed. Among 112 control cells, only one (1%) contained a monopolar CEN3 spot, and the remaining (99%) bioriented CEN3 ( Fig. 7d ). Furthermore, nearly all cells (99%) with CEN3 biorientation maintained stable separation of the sister pair over the entire imaging period ( Fig. 7d ). Therefore, the kinetochore biorientation defect in Hsk3-depleted cells directly supports predictions based on our in vitro experiments. Taken altogether, our findings suggest that oligomerization of the Dam1 complex is required for stable coupling of kinetochores to dynamic microtubule ends under tension in vivo . 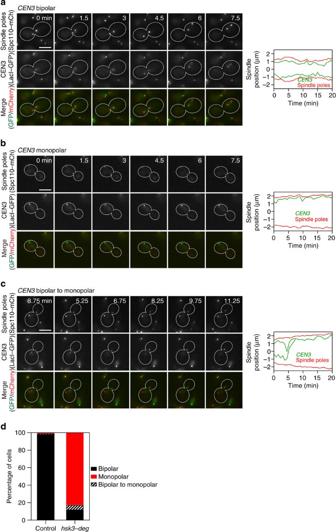Figure 7: The oligomerization-deficient Dam1 complex fails to support sister kinetochore biorientation. Representative time-lapse images ofhsk3–degroncells show the three classes ofCEN3behaviour: bioriented (a), monopolar (b) and biorientation failure (c). GFP and mCherry channels are shown separately and merged as inFig. 6. Scale bars, 5 μm; contrast was adjusted for visual clarity. Time stamps indicate elapsed time from the start of imaging. Shown to the right ina–care the plots of position versus time for spindle poles (red) andCEN3spots (green) from the corresponding time-lapse series. (d) Bar graph shows the percentage of cells in eachCEN3class for control (n=121) andhsk3–degron(n=168) cells. Figure 7: The oligomerization-deficient Dam1 complex fails to support sister kinetochore biorientation. Representative time-lapse images of hsk3–degron cells show the three classes of CEN3 behaviour: bioriented ( a ), monopolar ( b ) and biorientation failure ( c ). GFP and mCherry channels are shown separately and merged as in Fig. 6 . Scale bars, 5 μm; contrast was adjusted for visual clarity. Time stamps indicate elapsed time from the start of imaging. Shown to the right in a – c are the plots of position versus time for spindle poles (red) and CEN3 spots (green) from the corresponding time-lapse series. ( d ) Bar graph shows the percentage of cells in each CEN3 class for control ( n =121) and hsk3–degron ( n =168) cells. Full size image The Dam1 complex spontaneously assembles into oligomers in vitro , and forms rings that encircle microtubules. The functional consequences of oligomerization have remained unclear. One possibility is that oligomerization merely increases the avidity by allowing multiple Dam1 complexes to simultaneously contact the microtubule. Another non-mutually exclusive possibility is that oligomerization forms a structure with a specialized interaction with microtubule ends. For example, in its oligomeric ring conformation, the Dam1 complex is proposed to hook onto curled protofilaments at disassembling microtubule ends, thereby harnessing mechanical energy from the ‘conformational wave’ of microtubule disassembly [7] , [28] , [29] , [30] . However, oligomerization of the Dam1 complex has not been shown to be required for its functions either in forming direct attachments to dynamic microtubule ends in vitro , or in mediating these linkages at kinetochores in vivo . We addressed this question by using a version of the Dam1 complex that does not form oligomeric rings in vitro [14] . Here we show that this version of the Dam1 complex retains WT microtubule-binding behaviour at the level of single complexes, but lacks the ability to assemble into oligomers of any size, and is thus ‘Oligomerization-Deficient’ (Dam1 OD complex). In our optical trap assays, we found that oligomerization is required in vitro for the Dam1 complex to form microtubule attachments that are robust against applied mechanical loads. Due to the design of the assay, this function must be independent of binding avidity. Dam1 complexes were linked to the surface of polystyrene beads such that up to ~80 Dam1 complexes could simultaneously reach a microtubule end. This arrangement on the bead surface artificially imposes avidity; however, avidity alone is insufficient to rescue the defect of Dam1 OD complex in coupling to microtubule ends under tension. Therefore, oligomerization of the Dam1 complex contributes to the strength and processivity of microtubule attachments in a manner that is independent of binding avidity. Our findings support the possibility that oligomerization allows the Dam1 complex to form a ring that helps prevent its detachment from a flared microtubule end. We propose that this conformation is required at the kinetochore–microtubule interface in vivo , especially when kinetochores must sustain these linkages under tension during mitosis. We tested this hypothesis in vivo using an Hsk3–degron system to generate the oligomerization-deficient Dam1 complex in cells. We found that depletion of Hsk3 releases the oligomerization module of the Dam1 complex from its microtubule-binding module, indicating successful formation of the Dam1 OD complex in vivo . In Hsk3-depleted mitotic cells, bipolar centromere pairs collapsed to monopolar attachments. This microtubule attachment failure at one kinetochore of the sister pair can be explained directly by our in vitro results. The Dam1 OD complex is unable to mediate stable coupling to dynamic microtubule ends under tension. Following breakage, sister pairs remained attached in a monopolar state in vivo , consistent with the ability of the Dam1 OD complex to maintain attachments in the absence of tension in vitro . Thus, in the absence of oligomerization, the microtubule-binding ability of the Dam1 complex alone is insufficient to support stable kinetochore–microtubule attachment under tension in vivo . Our findings additionally suggest that oligomerization of the Dam1 complex can be regulated by controlling Hsk3 levels. Cells entering meiosis specifically suppress HSK3 expression among the genes encoding members of the Dam1 complex, and this regulation appears to promote the proper segregation of chromosomes during meiosis I (ref. 31 ). We speculate that the regulation of HSK3 might produce the Dam1 OD complex as the biologically relevant form of the Dam1 complex during meiosis I. Outside of fungal organisms, homologues of the Dam1 complex have not been identified; however, the Ska complex is a proposed functional equivalent in higher eukaryotes, and has been reported to form oligomeric structures in vitro [32] . Moreover, we and others have found that the human Ndc80 complex has evolved the ability to oligomerize [33] , [34] , [35] . Interestingly, the human Ndc80 complex is thought to oligomerize ‘longitudinally’ on microtubules, binding along individual protofilaments [33] . This form of oligomerization could provide functions distinct from those afforded by ‘lateral’ oligomerization (binding around the tube, as seen in Dam1 complex rings). The experiments presented here provide a framework to study how oligomerization contributes to kinetochore–microtubule coupling in other systems. Ultimately, we show that oligomerization is an important mechanism by which kinetochore components are coordinated to form a robust microtubule attachment site. Protein expression and purification All ten components of the S. cerevisiae Dam1 complex were co-expressed in Escherichia coli from a polycistronic vector [5] . The complex was affinity-purified using a C-terminal His 6 - or FLAG-tag on Spc34 and subjected to gel filtration, as previously described [8] , [9] , [12] . The expression vector was also modified to remove the gene encoding Hsk3; purification as carried out for the WT complex then yielded the six-protein oligomerization-deficient Dam1 complex, as previously reported [14] . For TIRF microscopy experiments, the Dam1 complex was tagged by fusion of GFP to the C-terminus of Dad1 [8] . The S. cerevisiae Ndc80 complex was expressed in E. coli , purified using a C-terminal His 6 -tag, and subjected to gel filtration, as reported previously [12] , [18] , [36] . Native kinetochore particles were purified from asynchronously growing S. cerevisiae cells using Dsn1-His 6 -FLAG (refs 10 , 11 ). Cells were grown in yeast peptone dextrose rich (YPD) medium [37] and extract was prepared by lysing cells in a blender in the presence of dry ice. Lysed cells were resuspended in buffer H (BH) (25 mM HEPES pH 8.0, 2 mM MgCl 2 , 0.1 mM EDTA, 0.5 mM EGTA, 0.1% NP-40, 150 mM KCl and 15% glycerol) containing protease and phosphatase inhibitors followed by ultracentrifugation at 98,500 g for 90 min at 4 °C. Beads conjugated with anti-FLAG antibodies were incubated with extract for 3 h with constant rotation, followed by three washes with BH containing protease inhibitors, phosphatase inhibitors and 2 mM dithiothreitol (DTT). Beads were further washed twice with BH-containing protease inhibitors. Associated proteins were eluted from the beads by gentle agitation of beads in elution buffer (0.5 mg ml −1 3 × FLAG peptide in BH with protease inhibitors) for 30 min at room temperature. Electron microscopy Sample preparation and imaging were performed essentially as described previously [12] . In brief, taxol-stabilized microtubules (36 nM polymerized tubulin) were incubated with 20 nM Dam1 WT complex or Dam1 OD complex. A 2-μl drop of sample was applied to a negatively charged carbon-coated copper grid (Electron Microscopy Sciences (EMS)). Grids were washed with BRB80 (80 mM PIPES, 120 mM K + , 1 mM MgCl 2 and 1 mM EGTA, pH 6.9) and then stained with 0.075% uranyl formate. Images were collected on a Spirit T12 (FEI) at × 52,000 magnification at the specimen level with 1 s exposure. TIRF microscopy Flow chambers were constructed and functionalized as reported previously [8] , [12] , [18] , [38] . Coverglass was adhered to a glass slide using double sticky tape, forming individual flow channels between two adjacent strips of tape. ‘Rigour’ kinesin was introduced and allowed to adsorb non-specifically to the glass, allowing the immobilization of taxol-stabilized microtubules on the coverslip. Single-molecule imaging experiments were carried out by incubating 5-40 pM Dam1 WT or Dam1 OD complex with Alexa-647-labelled microtubules. GFP and Alexa-647 fluorescence channels were simultaneously recorded using a custom TIRF imaging system [38] . In ‘tracer’ assays, GFP-tagged and unlabeled versions of the Dam1 complex were pre-mixed at a 1:100 ratio to a total concentration of 2 nM (Dam1 WT complex) or 20 nM (Dam1 OD complex) and subsequently incubated with microtubules. All TIRF assays were performed in BRB80 containing 1 mg ml −1 κ-casein, and supplemented with an additional 70 mM KCl and an oxygen scavenger system (200 μg ml −1 glucose oxidase, 35 μg ml −1 catalase, 25 mM glucose and 5 mM DTT). Single-particle tracking and analysis was performed using custom software (available upon request) developed in Labview (National Instruments) and Igor Pro (Wavemetrics) as reported previously [8] , [12] , [18] . Average binding densities of Dam1 WT and Dam1 OD complexes on microtubules ( Supplementary Fig. 2b ) were measured using the line scan function in ImageJ (NIH). Photo-bleaching experiments were carried out by non-specifically adsorbing GFP-tagged Dam1 complexes to the coverglass at a density of ~100 complexes per field of view (1,150 μm 2 ) and imaging under conditions identical to those used in single-molecule experiments. Automated analysis of single-step photo-bleach events was performed by fitting a heavy-side step function to records of brightness intensity over time (custom software developed in Labview, available upon request). Bootstrapping analysis was used to determine mean residence time and to estimate the error of the mean. Each residence time data set was randomly resampled with replacement 1,000 times. For both Dam1 WT and Dam1 OD complexes, the means of the resampled data sets formed normal distributions. Gaussian fits to these distributions yielded estimates of mean residence time, and the Gaussian width was used as an estimate of the error. Protein size analysis Size-exclusion chromatography was carried out using a HiLoad Superdex 16/60 prep grade column (GE Healthcare) equilibrated in Dam1 purification buffer (500 mM NaCl, 50 mM phosphate, pH 6.9). The column was calibrated using BSA, catalase, ferritin and thyroglobulin as protein size standards. For velocity sedimentation analysis, a 90-μl sample of 2 μM Dam1 WT or Dam1 OD complex was loaded onto a 1-ml 8–32% sucrose gradient made in Dam1 purification buffer; BSA, catalase and aldolase were used as protein size standards. Optical trap-based bead motility assays Streptavidin-coated 0.44-μm polystyrene beads (Spherotech) were functionalized with biotinylated anti-His 5 antibody (Qiagen) and decorated with Dam1 complexes via recognition of the His 6 -tag on the C terminus of Spc34. Incubation of 11 pM beads and 20 nM Dam1 complex (for ~1 h at 4 °C) yielded a surface density of ~2,000 complexes per bead. In this arrangement, we estimate that up to ~80 Dam1 complexes can simultaneously reach from the bead surface to the microtubule end [18] . Bead decoration was performed in a total volume of 60 μl incubation buffer (BRB80 containing 8 mg ml −1 BSA and 1 mM DTT). Any remaining Dam1 complex not bound to the bead surface was removed by pelleting the beads (16,000 g for 10 min at 4 °C) and washing with ~200 μl incubation buffer. Beads were returned to the original incubation volume by pelleting (16,000 g for 10 min at 4 °C) and resuspending in 60 μl incubation buffer. Beads coated with Ndc80 complex were prepared in the same manner as described for the Dam1 complex. Kinetochore particles were diluted such that the concentration of Dsn1 was ~0.4 ng ul −1 , and then incubated with 6 pM beads for ~1 h at 4 °C, as described previously [10] , [11] . Flow chambers were prepared to immobilize GMPCPP-stabilized microtubule seeds on the coverglass, as previously described [17] , [34] . Beads were introduced into the flow chamber in assay buffer (BRB80 containing 8 mg ml −1 BSA, 1 mg ml −1 κ-casein, 1 mM DTT, 1 mM GTP and 1.4 mg ml tubulin) supplemented with an oxygen scavenging system (250 μg ml −1 glucose oxidase, 30 μg ml −1 catalase and 30 mM glucose). Dynamic microtubule extensions were assembled by the addition of free tubulin dimers onto the coverglass-bound GMPCPP-stabilized microtubule seeds. A custom optical trap instrument [17] was used to capture and manipulate beads, and to apply force to the attachments between the Dam1 complex and dynamic microtubule ends. Rupture force experiments were performed essentially as described previously [10] , [11] , [12] . Beads were initially attached to microtubules and subjected to a 2.4-pN constant ‘test’ force in the direction of microtubule growth. Beads were required to track microtubule growth over a distance of ~100–500 nm to ensure end-on attachment. After satisfying the test phase, the applied force was increased at a constant rate of 0.25 pN s −1 until bead detachment. Records of force versus time collected during the experiment were used to determine the rupture force, which was marked as the maximum force sustained by the attachment during each event. Some rupture force assays included FLAG-tagged Dam1 complex added free in solution along with the beads; this free Dam1 complex was supplied in the assay buffer. Constant force experiments were also carried out as previously reported [9] , [18] , [19] . Briefly, beads were attached to assembling microtubule ends, and 2.4 pN was applied continuously (in the direction of microtubule growth) throughout rounds of microtubule assembly and disassembly. Upon bead detachment, microtubule tip state was determined visually during the experiment and confirmed during subsequent analysis using traces of bead position versus time. Attachment lifetime and microtubule dynamic rates were also measured from bead position traces using custom software (available upon request) developed in Igor Pro. For experiments performed in the absence of applied force, beads were tracked by differential interference contrast imaging as previously described [19] . Beads were bound to the microtubule lattice, and a secondary laser was used to induce microtubule disassembly by ablation of the plus end, as reported previously [12] , [34] . Attachment lifetime was measured from video recordings and was defined as the period over which recognizable disassembly-driven motility occurred. Yeast culture and live-cell imaging Strains used in this study are listed in Supplementary Table 1 and are derivatives of SBY3 (W303). NUF2–GFP and SPC110-mCherry (ref. 1 ), pCUP1-GFP12-LacI12 and CEN3::33LacO (ref. 39 ), TUB1-GFP (ref. 40 ) and OsTIR1-9myc constructs [22] were described previously. ASK1–YFP was created as described [41] . HSK3-3V5-IAA7, DAM1-3V5-IAA7 and DAD1-GFP were constructed by PCR-based methods as reported previously [42] . Primer sequences for strain constructions are available upon request. Auxin-inducible degron alleles were generated by fusing the protein of interest with 3V5-IAA7. Plasmids for 3V5-IAA7 fusion were kindly provided by Dr Leon Chan (UC Berkeley). Cultures were grown at 30 °C in YPD to ~30–60 Klett. The auxin-inducible degron system [22] was activated by addition of 0.5 mM auxin to the growth medium (YPD+auxin). Cells were mounted on agar pads as described previously [43] or in a CellAsic (Millipore) microfluidics device and imaged using a DeltaVision system (Applied Precision) fitted with an IX70 inverted fluorescence microscope (Olympus), a Uplan APO × 100 objective (1.35 NA) and a CoolSnap HQ camera (Photometrics). For localization experiments, asynchronously growing cells were collected for imaging on agar pads at designated timepoints after the addition of auxin. Exposures of 0.3 s were recorded for Dad1–GFP or Ask1–YFP in each of nine 0.5-μm optical sections. Automated spot detection was performed using custom Matlab-based software, Fluorcal [44] , available upon request. Cells were counted visually using differential interference contrast images taken in the same field of view. Spindle morphology was assessed in asynchronously growing cultures after treatment with auxin for 2 h. Tub1–GFP and Spc110–mCherry were imaged as described for Dad1–GFP and Ask1–YFP. Spindles were considered broken if Tub1–GFP fluorescence was not oriented along the spindle axis. Kinetochore biorientation was imaged in synchronized cells using the CellAsic system. Asynchronous cells (~30 Klett) were loaded into the microfluidics chamber and grown in YPD+6 μM α-factor medium for 2 h. Auxin was then introduced by exchanging to YPD+6 μM α-factor+0.5 mM auxin medium for 1 h. Cells were subsequently released from α-factor into YPD+auxin medium and imaged in three 1.5-μm optical sections at 7.5-min intervals from the time of release. Nuf2–GFP and Spc110–mCherry were imaged with exposures of 0.1 s and 0.3 s, respectively. For each cell, a single representative frame in which both spindle poles were in good focus was used to generate a spindle profile. Spindle profiles were generated from maximum intensity projections of the GFP and mCherry channels with the ImageJ line scan tool. Automated analysis was performed on each spindle profile using custom software developed in Igor Pro, available upon request. Spindle poles were located using Gaussian fitting, and the spindle midzone was defined as the midpoint between the two poles. GFP fluorescence intensity was then integrated in each half spindle (as defined by the spindle midzone) to obtain the ‘kinetochore intensity’ associated with each spindle pole. The kinetochore intensity ratio was then determined as the larger kinetochore intensity divided by the smaller; by definition, this ratio is always ≥1. Average spindle profiles were obtained by normalizing spindle length: the spindle pole associated with the larger kinetochore intensity was defined as position 0, and the opposite spindle pole as position 1. GFP intensity was binned in increments of 0.05 along the normalized spindle axis and averaged across all measured spindles. In biorientation experiments, CEN3 was visualized using LacI–GFP bound to a lacO array adjacent to the centromere. LacI–GFP is under control of the pCUP1 promoter and imaged using uninduced conditions, with media made from yeast nitrogen base lacking copper (ForMedium). Auxin was added to asynchronous cultures, and live cells were imaged on agar pads at 45-s intervals for up to 30 min. LacI–GFP and Spc110–mCherry were imaged with 0.3 s exposures in nine 0.5-μm optical sections, as described above for Dad1–GFP. Biorientation was scored manually after the experiment for all cells in which both spindle poles remained in focus throughout the observation period. Position versus time traces were obtained from four-dimensional automated spot tracking applied to the mCherry and GFP channels using Imaris (Bitplane). How to cite this article : Umbreit, N. T. et al . Kinetochores require oligomerization of Dam1 complex to maintain microtubule attachments against tension and promote biorientation. Nat. Commun. 5:4951 doi: 10.1038/ncomms5951 (2014).